Visible-light-enhanced gating effect at the LaAlO3/SrTiO3interface Electrostatic gating field and light illumination are two widely used stimuli for semiconductor devices. Via capacitive effect, a gate field modifies the carrier density of the devices, while illumination generates extra carriers by exciting trapped electrons. Here we report an unusual illumination-enhanced gating effect in a two-dimensional electron gas at the LaAlO 3 /SrTiO 3 interface, which has been the focus of emergent phenomena exploration. We find that light illumination decreases, rather than increases, the carrier density of the gas when the interface is negatively gated through the SrTiO 3 layer, and the density drop can be 20 times as large as that caused by the conventional capacitive effect. This effect is further found to stem from an illumination-accelerated interface polarization, an originally extremely slow process. This unusual effect provides a promising controlling of the correlated oxide electronics in which a much larger gating capacity is demanding due to their intrinsic larger carrier density. The two-dimensional electron gas (2DEG) at the heterointerfaces between complex oxides has received attention in recent years because of its implementation for novel physics and prospective applications [1] , [2] , [3] , [4] , [5] , [6] , [7] , [8] , [9] , [10] , [11] , [12] , [13] . The 2DEG confined to the LaAlO 3 /SrTiO 3 (LAO/STO) interfaces is a representative system that has been extensively studied, and exotic properties including two-dimensional superconductivity [3] , magnetism [5] , enhanced Rashba spin–orbital coupling [6] and strong electrical field effect [4] , [7] , [8] , [9] , [10] , [11] , [12] , [13] have been observed. Among these, the field effect is particularly interesting. As already demonstrated, the transport behaviour can be tuned by a gate field across STO or LAO, undergoing a metal-to-insulator transition [9] or a tunable superconducting transition [3] , [13] . On the other hand, a dramatic modification of the interfacial conductivity can also be gained by depositing polar molecules or charges above the LAO layer [7] , [8] . Obviously, gating effect has shown its potential in unravelling the emergent phenomena at complex oxide interfaces. However, the electrical field effect for the complex oxide 2DEG is much more complicated than for the conventional semiconductor devices. In addition to electrons, there are many other factors such as ionic defects, trapped charges or ferroelectric instabilities in the system that can be severely affected by the applied electric field. As a consequence, significant hysteresis of interfacial conductivity can occur when cycling electrical bias through the STO crystal [9] or scanning a biased tip across the LAO layer, the latter leads to conducting nanowires persisting for days [10] , [11] . A few recent reports [9] , [14] even show that the field effect actually exhibits two steps: a fast process is followed by an extremely slow process that usually lasts for thousands of seconds but owns a tuning ability comparable to or even stronger than the fast one [14] . While the slow process yields additional freedom in controlling the physical properties of the 2DEG, its slow nature makes it hard to be exploited in any practical devices but causes an adverse influence to the reproducibility. In this work, we report on a remarkable effect produced by combined electrical and optical stimuli for the 2DEGs at both amorphous and crystalline LAO/STO heterointerfaces (a-LAOSTO and c-LAO/STO, respectively). We found that an illumination of visible light drives the slow field-induced resistance growth into a great jump far beyond the scope of normal field effect, markedly enhancing the ability of the gate field to modulate charge carriers. The present work clearly demonstrates the mutual reinforcement of the effects of electrical gating and light illuminating on complex oxide interfaces. Illumination-accelerated gating effect Details for sample fabrication and resistive measurements are described in the Methods. 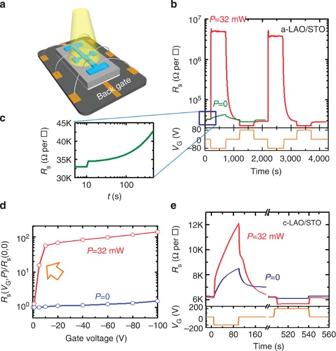Figure 1:Resistive responses to electrical and optical stimuli of the LAO/STO interface. (a) A sketch of the experimental set-up. (b) Sheet resistance of a-LAO/STO, recorded in the presence/absence of a light ofP=32 mW (λ=532 nm) whileVGswitches among −80, 0 and +80 V. (c) Enlarged view of the two-step feature ofRSwithout light illumination. (d) Gate dependence of normalized sheet resistance,RS(VG,P)/RS(0,0), recorded at the time of 300 s after the application ofVG. Arrow marks theRScorresponding toVG=−5 V. (e) Sheet resistance of c-LAO/STO, recorded in the presence/absence of a light ofP=32 mW (λ=532 nm) asVGswitches among −200, 0 and +200 V. All measurements were conducted at room temperature. Figure 1 shows the typical resistive responses of our devices to electrical and optical stimuli. As schemed in Fig. 1a , a gate voltage, V G , between −100 V and 100 V was applied to the back gate of STO while the a-LAO/STO interface was grounded and the sheet resistance, R S , was recorded in the presence/absence of a light illumination. In all cases, the leakage current (<7 nA) was much lower than the in-plane current applied for resistive measurements, 1 μA ( Supplementary Fig. 1 ). As shown in Fig. 1b,c , without illumination, the application of a V G =−80 V yields two distinct processes marked respectively by a slight jump and a followed steady increase of R S . The first minor jump is the normal gating effect, stemming from the field-induced charge density change in the backgate–interface capacitor. The latter process is extremely slow, lasting for >2,000 s without saturation and produces an R S increase much larger than the first jump. This process can be well described by the Curie–von Schweidler law R S ∝ ( t − t 0 ) α , which implies a wide distribution of the energy barriers that impede the carrier depletion (see Supplementary Fig. 2 ) [15] . Figure 1: Resistive responses to electrical and optical stimuli of the LAO/STO interface . ( a ) A sketch of the experimental set-up. ( b ) Sheet resistance of a-LAO/STO, recorded in the presence/absence of a light of P =32 mW ( λ =532 nm) while V G switches among −80, 0 and +80 V. ( c ) Enlarged view of the two-step feature of R S without light illumination. ( d ) Gate dependence of normalized sheet resistance, R S ( V G , P )/ R S (0,0), recorded at the time of 300 s after the application of V G . Arrow marks the R S corresponding to V G =−5 V. ( e ) Sheet resistance of c-LAO/STO, recorded in the presence/absence of a light of P =32 mW ( λ =532 nm) as V G switches among −200, 0 and +200 V. All measurements were conducted at room temperature. Full size image Remarkably, such a field effect is significantly modified by light illumination. Aided by a light of 32 mW ( λ =532 nm), as shown by the red curve in Fig. 1b , gate field drives R S into a sudden jump to a steady state of 200-fold resistance, that is, the slow process has been markedly accelerated by light illumination, and this change is reversible for the repeated on–off operations of the gate field. As summarized in Fig. 1d , a light of 32 mW pushes the R S ( V G =−100 V, P )/ R S (0,0) ratio from ~1.2 to ~202, amplifying the gating effect by ~170-fold. Moreover, even a V G as low as −5 V can cause a 17-fold R S growth (marked by an arrow). This bias is only one-tenth of that usually required to get comparable effect using a backgate without light [9] , [16] . The gating effect of positive V G was also enhanced by illumination but it is relatively weak (see Fig. 1b and Supplementary Figs 3 and 4 ). Similar illumination-enhanced gating effect is also observed in c-LAO/STO ( Fig. 1f ), suggesting that it is a quite universal phenomenon, independent of the characteristics of the electronic transport of the interface (it is semiconducting for a-LAO/STO and metallic for c-LAO/STO; refer to Supplementary Fig. 5 ) and the crystal structure of the LAO overlayer (crystalline or amorphous). Carrier density tuning beyond capacitive effect To gain a further understanding of this illumination effect, we examined the sheet carrier density, n S , by Hall measurement. From the linear R xy – H relation in Fig. 2a , the initial n S can be deduced, and it is ~7 × 10 12 cm −2 , where R xy is the Hall resistance. There are no detectable changes in the R xy – H dependence measured immediately after the application of a | V G |=100 V, indicating that the change in carrier density is tiny. It is consistent with the result deduced from the capacitance data in Fig. 2c , for P =0, which is only ~4% of the initial n S , where C a-LAO/STO is the capacitance of the backgate–interface capacitor, e is the electron charge and S≈ 5 mm 2 is the interface area. In contrast, in a light of P =6 mW (the highest intensity available for our Hall-effect measurement system), a V G =−100 V reduces the n S from ~7.0 × 10 12 to ~1.3 × 10 12 cm −2 ( Fig. 2b ) and the mobility from ~25.8 to ~1.2 cm 2 V −1 s −1 (deduced from the data in Fig. 2b ). This extraordinarily large Δ n S is confirmed by the sudden C a-LAO/STO drop shown in Fig. 2c for V G <−20 V and P =32 mW, which suggests the exhaustion of sheet carriers. A large Δ n S (~1.1 × 10 13 cm −2 for a V G of −200 V) is also detected in illuminated c-LAO/STO ( Supplementary Fig. 6 ). However, the illumination enhancement is almost absent when the interface is positively gated. In this case, as shown by the data of V G =0 (black) and 100 V (magenta) in Fig. 2a , Δ n S increases slightly and can be ascribed to the illumination-generated extra photocarriers. 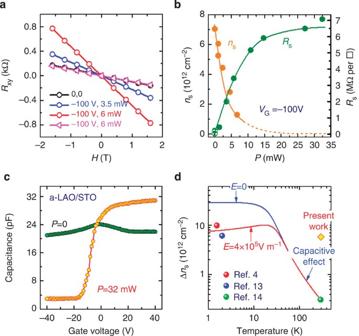Figure 2: Hall effect and capacitance measurements. (a) Hall resistance,Rxy, of a-LAO/STO measured with an in-plane current of 10 μA under different gating/illuminating conditions. Without light illumination the data forVG=−100 V cannot be distinguished from those forVG=0, and therefore are not shown here. (b) Carrier density and sheet resistance as functions of light power, acquired under a fixedVGof −100 V. Solid lines are guides for the eye. Dashed line is the extrapolatednS–Prelation. (c) Capacitance,Ca-LAO/STO, of a-LAO/STO as a function of gate voltage, measured under the a.c. amplitude of 0.5 V and frequency of 5 kHz. Labels in the figure denote light power (λ=532). (d) Carrier density change produced by capacitive effect, calculated by ΔnS=ε0εVG/dadopting the permittivity under a constant electrical field marked beside the curve andVG=100 V. Symbols are experimental values for |VG|=100 V extracted from literature, as indicated in the figure. Figure 2: Hall effect and capacitance measurements. ( a ) Hall resistance, R xy , of a-LAO/STO measured with an in-plane current of 10 μA under different gating/illuminating conditions. Without light illumination the data for V G =−100 V cannot be distinguished from those for V G =0, and therefore are not shown here. ( b ) Carrier density and sheet resistance as functions of light power, acquired under a fixed V G of −100 V. Solid lines are guides for the eye. Dashed line is the extrapolated n S – P relation. ( c ) Capacitance, C a-LAO/STO , of a-LAO/STO as a function of gate voltage, measured under the a.c. amplitude of 0.5 V and frequency of 5 kHz. Labels in the figure denote light power ( λ =532). ( d ) Carrier density change produced by capacitive effect, calculated by Δ n S = ε 0 εV G / d adopting the permittivity under a constant electrical field marked beside the curve and V G =100 V. Symbols are experimental values for | V G |=100 V extracted from literature, as indicated in the figure. Full size image According to the capacitor model, the depleted carrier density by a negative V G is Δ n S = ε 0 ε | V G |/ d , where ε is the relative dielectric constant of STO and d is the thickness of STO. Adopting the ε values in ref. 17 , the tuned carrier density by the capacitive effect can be calculated. As shown in Fig. 2d , the illumination-enhanced gating effect is much stronger than the simple gating effect that is always well described by the conventional capacitive effect. This result strongly suggests that additional mechanisms are at work under light illumination. To explore the origin of this unusual illumination-enhanced asymmetric gating effect, we examined the dependence of the field effect on light wavelength, λ . As shown in Fig. 3a , the tuned value of R S drops rapidly as λ increases from 532 to 980 nm, suggesting that the photoexcitation of trapped electrons play a key role in the observed effect, although, counter-intuitively, the photoexcitation process significantly decreases, rather than increases, n S . Furthermore, a strong-to-weak crossover of the illumination effect occurs at λ ~850 nm ( Fig. 3b , V G =−20 V), corresponding to a photon energy of ~1.4 eV. This value coincides well with the reported deep oxygen vacancy states with one trapped electron in STO [18] , [19] . 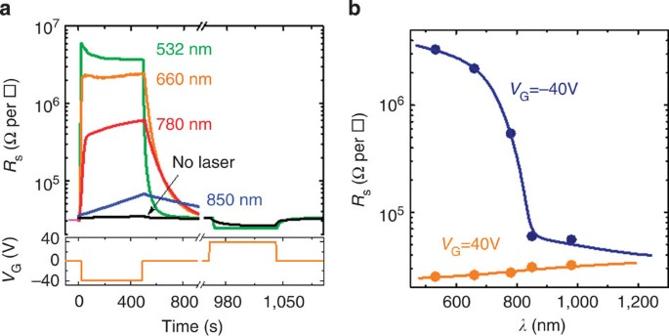Figure 3: Field effect measured in different lights. (a) Sheet resistance of a-LAO/STO corresponding to the field switching between on and off states, collected at a constant light power (32 mW) but different wavelengths. For clarity, only the data forP=0 andλ=532 nm are shown forVG=+40 V. (b) Sheet resistance as a function of light wavelength, acquired at the time of 200 s forVG<0 and 1,000 s forVG>0. Solid lines are guides for the eye. All the measurements were conducted at room temperature. Figure 3: Field effect measured in different lights. ( a ) Sheet resistance of a-LAO/STO corresponding to the field switching between on and off states, collected at a constant light power (32 mW) but different wavelengths. For clarity, only the data for P =0 and λ =532 nm are shown for V G =+40 V. ( b ) Sheet resistance as a function of light wavelength, acquired at the time of 200 s for V G <0 and 1,000 s for V G >0. Solid lines are guides for the eye. All the measurements were conducted at room temperature. Full size image Gating-induced and illuminating-enhanced lattice polarizations As reported, oxygen vacancies (V O ) tend to pile up close to the STO surface [20] , [21] , [22] , [23] and drift slowly under electrical field [24] . A recent study has shown that the electromigration of oxygen vacancies can lead to a polarity-asymmetric interface polarization [25] , which was built up in >20 h under a strong field. This slow buildup of the polar phase is reminiscent of the slow gating process observed when only the electrical field is applied ( Fig. 1b ). It is therefore possible that the illumination-enhanced gating effect is triggered by the acceleration of the establishment process of this interface phase. Direct evidence comes from Fig. 4 , where a field-induced structural deformation of a-LAO/STO is indicated by X-ray diffraction. 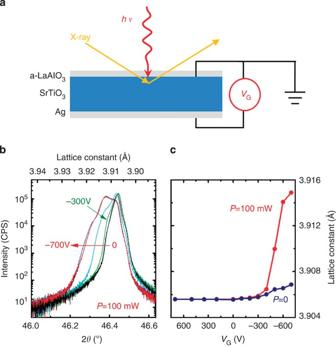Figure 4: Light illumination acceleration of the field-induced structural deformation of STO. (a) Experiment set-up for the structural measurements of a-LAO/STO with simultaneously applied light illumination and gate field. (b) X-ray diffraction patterns of the 002 reflection of STO measured after a waiting time of 10 min upon the simultaneous application of light illumination (P=100 mW,λ=532 nm) and gate biases. The two shoulders developed on the low-angle side of the 002 reflection mark the lattice expansion in the near interface region of a-LAO/STO. Labels besides the curves indicate gate voltage. The total time required for eachθ−2θscanning is ~10 min. (c) A comparison of the lattice constants obtained with and without light illumination. The acceleration of the field-induced structural deformation by photoexcitation can be clearly seen. Solid lines are guides for the eye. Figure 4a is the experimental set-up for structural measurements. Figure 4b is the θ −2 θ diffraction patterns, and Fig. 4c is the deduced out-of-plane lattice constant of STO, as a function of electric biases. When illuminated, as shown by Fig. 4b , a low-angle shoulder of the 002 reflection of STO emerges and develops above V G ≈−300 V, indicating an out-of-plane lattice expansion. However, no structural changes are observed up to the gate bias of −700 V without illumination. This result indicates that the light illumination indeed helps the gate field in inducing a structural deformation. As revealed by the previous work [25] , the lattice expansion of STO is a signature of interface polarization [25] . The structural distortion could not be a thermal effect as it continues to remain once it has appeared even after the sample is shaded from light, and the illumination alone produces no effect on structure (see Supplementary Fig. 7 ). Notably, the threshold V G for structural deformation is much higher than that for remarkable resistance tuning. It may be a consequence of uneven gating due to preferential carrier exhaustion around electrode, which confines gate field to the close proximity of the electrode. The uneven tuning can be sensed by sheet resistance since the latter is susceptible to local environment but not by X-ray diffraction unless V G is so high that the strongly gated area has well outward extension. We also performed the X-ray diffraction measurements for a Ti (30 nm)/STO/Ti (200 nm) capacitor structure and observed a similar lattice expansion ( Supplementary Fig. 7 ). Without uneven gating, here the interface phase appears under a V G below −200 V. Corresponding to the emergence of interface phase, forbidden shifts in Raman spectra were detected, implying an inversion symmetry breaking ( Supplementary Fig. 8 ). These results strongly suggest that light illumination has greatly accelerated the formation of the interface polarization phase. Figure 4: Light illumination acceleration of the field-induced structural deformation of STO. ( a ) Experiment set-up for the structural measurements of a-LAO/STO with simultaneously applied light illumination and gate field. ( b ) X-ray diffraction patterns of the 002 reflection of STO measured after a waiting time of 10 min upon the simultaneous application of light illumination ( P =100 mW, λ =532 nm) and gate biases. The two shoulders developed on the low-angle side of the 002 reflection mark the lattice expansion in the near interface region of a-LAO/STO. Labels besides the curves indicate gate voltage. The total time required for each θ −2 θ scanning is ~10 min. ( c ) A comparison of the lattice constants obtained with and without light illumination. The acceleration of the field-induced structural deformation by photoexcitation can be clearly seen. Solid lines are guides for the eye. Full size image On the basis of the above analyses, we can present a scenario for the illumination-enhanced gating effect. As schemed in Fig. 5a , the oxygen vacancy concentration at the LAO/STO interface is considerably high due to the outward oxygen ion diffusion from the STO substrate during the deposition of the LAO overlayer, and the resulted electron doping leads to the 2DEG at the a-LAO/STO interface [21] , [22] , [23] and might also contribute to the conduction of the c-LAO/STO interface. Without illumination, negative bias only slightly polarizes the interface region of STO ( Fig. 5b ), yielding the slow R S growth following the first sudden R S jump ( Fig. 1c ). Light illumination accelerates interface polarization by enhancing the electromigration of oxygen vacancies, probably by exciting the trapped electrons in deep oxygen vacancy states ( Fig. 5c ). This polarization yields an extra tuning to n S and a weakening of the interfacial confining well of 2DEG. These two effects markedly reduce n S , amplifying the gating effect. 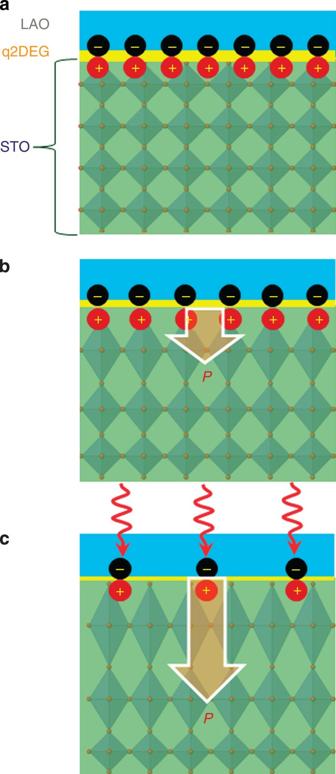Figure 5:Migration of oxygen vacancies under electrical field and light illumination. (a) The content of oxygen vacancy (marked by circled plus symbols) is considerably high at the LAO/STO interface due to the outward diffusion of oxygen ions from STO, resulting in electron doping (marked by circled minus symbols) and thus the 2DEG at the a-LAO/STO interface. The oxygen vacancy here may be mainly in the state with one deeply trapped electron,, the most favourable state when vacancy content is high27,28,29,30. (b) The inward migration of these interface oxygen vacancies under negative gate biases will induce an interface polarization phase25. Owing to the low mobility ofs, however, it is difficult for the gate field alone to cause significant vacancy migration. As a result, a negative bias only slightly polarizes the interface region of STO, yielding a very weak tuning to sheet carriers. (c) Light illumination excites the trapped electron in, transitingthe latter into thestate that is much more susceptible to external field. In this manner, it accelerates the electromigration of oxygen vacancies, thus the building up of the polarization phase that causes a strong extra tuning to sheet carriers. Figure 5: Migration of oxygen vacancies under electrical field and light illumination . ( a ) The content of oxygen vacancy (marked by circled plus symbols) is considerably high at the LAO/STO interface due to the outward diffusion of oxygen ions from STO, resulting in electron doping (marked by circled minus symbols) and thus the 2DEG at the a-LAO/STO interface. The oxygen vacancy here may be mainly in the state with one deeply trapped electron, , the most favourable state when vacancy content is high [27] , [28] , [29] , [30] . ( b ) The inward migration of these interface oxygen vacancies under negative gate biases will induce an interface polarization phase [25] . Owing to the low mobility of s, however, it is difficult for the gate field alone to cause significant vacancy migration. As a result, a negative bias only slightly polarizes the interface region of STO, yielding a very weak tuning to sheet carriers. ( c ) Light illumination excites the trapped electron in , transitingthe latter into the state that is much more susceptible to external field. In this manner, it accelerates the electromigration of oxygen vacancies, thus the building up of the polarization phase that causes a strong extra tuning to sheet carriers. Full size image Effect of light illumination on the electromigration of oxygen vacancies in STO can be identified from the transient leakage current recorded under a constant d.c. bias. As well established, prior to resistance degradation, a broad current peak will appear when the V O s in the near region of the anode reach cathode [25] , [26] . As shown by the Supplementary Fig. 9 , for the STO biased by a V G of −600 V, the current peaks at ~580, ~115 and ~16 min for the light power of 0, 40 and 100 mW, that is, illumination indeed accelerates the migration of oxygen vacancies. As revealed by ref. 25 , the polarization will disappear in several seconds after removing the external field. This is consistent with our observation that R S quickly drops back when the gate bias is removed ( Fig. 1b ). No additional tuning is observed under positive gate fields since there are no structural changes ( Fig. 4b ). In conclusion, our present work has revealed a unique control of the 2DEG confined at the LAO/STO interface with complementary electric and light stimuli. The principle proven here could be extended to a wide variety of complex oxide systems with ferroelectric instabilities, pioneering a new avenue for the resistive tuning of oxide interfaces. Sample fabrication The samples a-LAO/STO were prepared by depositing an amorphous LAO layer, ~12 nm in thickness, on TiO 2 -termined (001)-STO substrates (3 × 5 × 0.5 mm 3 ) using the pulsed laser (248 nm) ablation technique. In the deposition process, the substrate was kept at ambient temperature and the oxygen pressure at 10 −3 mbar. The fluence of the laser pulses was 1.5 J cm −2 and the repetition rate was 1 Hz. The target–substrate separation was 4.5 cm. A shadow mask was employed to get the Hall-bar-shaped samples. For comparison, sample c-LAO/STO with a crystalline LAO overlayer (4 unit cells in thickness) was also prepared at a temperature of 800 °C and the oxygen pressure of 10 −5 mbar. The fluence of the laser pulses was 0.7 J cm −2 and the repetition rate was 1 Hz. After deposition, the sample was in situ annealed in 200 mbar of O 2 at 600 °C for 1 h and then cooled to room temperature in the same oxygen pressure. The detailed procedures for sample preparation can be found in ref. 21 for amorphous overlay and in ref. 7 for crystalline overlayer. Measurements Ultrasonic Al wire bonding (20 μm in diameter) was used for electrode connection. Four-probe technique was adopted for resistance measurements. The four welding spots were well aligned and the separation between the neighbouring spots was ~0.4 mm. The formula of R S ≈( L / W ) R was adopted for the convention of four-probe resistance to sheet resistance, where L and W are, respectively, the long and wide dimensions of the measured plane. Transverse electrical field was applied to STO through an Ag electrode underneath STO and the LAO/STO interface was grounded. The direction from substrate to interface was defined as positive. The applied current for resistance measurements was 1 μA. Lasers with the wavelengths between 532 and 980 nm were used in the present experiments. The spot size of the light was ~0.4 mm in diameter, focusing on the space between two inner Al wires. Under the gate voltage of −100 V, the leakage current was ~0.7 nA without illumination and at most ~7 nA under light illumination (refer to Supplementary Fig. 1 ). The crystal structure of the gated c-LAO/STO was measured by a Bruker diffractometer (D8 Discover, Cu K α radiation), using the X-ray parallelized and monochromatized by an asymmetric Ge 2202-Bounce monochromator. Capacitance was measured by the Precision Impedance Analyzer (Agilent 4294 A), adopting the a.c. amplitude of 0.5 V and the frequencies of 100 Hz and 5 kHz. The data were recorded after an interval of 60 s after the application of V G and the whole measurement from −40 V to 40 V takes 180 s. All data, except for the R S – T relations, were acquired at ambient temperature. How to cite this article: Lei, Y. et al . Visible-light-enhanced gating effect at the LaAlO 3 /SrTiO 3 interface. Nat. Commun. 5:5554 doi: 10.1038/ncomms6554 (2014).